Experience enhances gamma oscillations and interhemispheric asymmetry in the hippocampus Gamma oscillations are implicated in higher-order brain functions such as cognition and memory, but how an animal’s experience organizes these gamma activities remains elusive. Here we show that the power of hippocampal theta-associated gamma oscillations recorded during urethane anesthesia tends to be greater in rats reared in an enriched environment than those reared in an isolated condition. This experience-dependent gamma enhancement is consistently larger in the right hippocampus across subjects, coinciding with a lateralized increase of synaptic density in the right hippocampus. Moreover, interhemispheric coherence in the enriched environment group is significantly elevated at the gamma frequency. These results suggest that enriched rearing sculpts the functional left–right asymmetry of hippocampal circuits by reorganization of synapses. Gamma (25–140 Hz) rhythms serve to synchronize neurons and form cell assemblies in mammalian cortical structures [1] . In rodent hippocampus, gamma oscillations appear in the local field potential (LFP) during theta states [2] , which occur during active exploration and rapid eye movement sleep. Hippocampal place cells that encode similar spatial positions in an environment tend to discharge within the same gamma cycles [3] , supporting the idea that gamma oscillations are a mechanism coordinating cell assemblies (for example, Lisman and Idiart [4] ). Despite mounting studies of gamma oscillations as a temporal code of spatial information, how animals’ experience organizes the gamma activity remains largely unaddressed. Here we show that the experience of an enriched environment enhances gamma oscillations in CA1 stratum radiatum ( s.r. ) of the rat hippocampus. The magnitude of the gamma-amplitude enhancement is greater on the right side, correlating with an increase of local synaptic density. Moreover, a significant elevation of interhemispheric gamma oscillation synchrony is observed. These gamma oscillation changes are attenuated by chronic administration of an NMDA ( N -methyl- D -aspartate) receptor (NMDAR) antagonist, ketamine. Together, these results indicate that enriched rearing sculpts the functional left–right asymmetry of hippocampal circuits by reorganization of synapses. Experience-dependent laterialization of gamma oscillations Exposing animals to enriched environments with various tactile, spatial and social experiences for 3–4 weeks is known to improve the animals’ ability to perform hippocampus-dependent behavioural tasks [5] , [6] . To study how experience sculpts hippocampal neuronal dynamics, we compared Long-Evans rats reared in isolation in standard cages (ISO) with those reared in groups in enriched environments (ENR) ( Fig. 1a ). 3.5–4.5 weeks after weaning, rats were anesthetized with urethane (1.6 g kg −1 ), and 16-channel linear silicon probes were used to record bilaterally in the CA1 region of the hippocampus ( Fig. 1b , Supplementary Fig. S1 ). We employed a level of anesthesia in which theta and non-theta periods alternated spontaneously. We then used an algorithm that automatically extracted theta periods (see methods) and analyzed gamma oscillations during these times. The long-term gamma power was stable during theta episodes ( Supplementary Fig. S2 ), and simply by eye, it was clear that the amplitude of gamma oscillations in the ENR group was larger than that of ISO ( Fig. 2a ). As slow and fast gamma oscillations in CA1 are generated, respectively, in s.r. and stratum lacunosum moleculare ( s.l-m. ) [7] , [8] , we analyzed the gamma oscillation changes in the two frequency bands separately ( Fig. 2b ). For slow gamma power (30–45 Hz), power spectral analysis revealed an average increase of 103% (ISO: 693.9±234.8 μV 2 , N ISO =10; ENR: 1409±434.3 μV 2 , N ENR =10) in the right hemisphere of the ENR rats, and there was a tendency for an increase on the left side as well (51.1% increase, ISO: 757.9±281.7 μV 2 , ENR 1151±241.4 μV 2 ; Fig. 2c ). Two-way analysis of variance (ANOVA) indicated a significant interaction between the environmental effects and the side of the hippocampus on the gamma power (F(1, 18)=8.2000, P =0.0103)). The main effect of the environment or the laterality was less influential than the combined effect (F(1, 18)=2.217, P =0.154; F(1, 18)=3.039, P =0.0984, respectively). For fast gamma (55–90 Hz), the increase in power was smaller (left, ISO: 150.6±29.86 μV 2 versus ENR: 170.7±23.66 μV 2 , 15.4% increase; right, ISO: 138.5±26.26 μV 2 versus ENR: 201.6±26.95 μV 2 , 45.6% increase; F(1,18)=1.327, P =0.264 for the environment; F(1,18)=1.954, P =0.179 for the side), however, once again the ANOVA showed a significant interaction of the environment and hemisphere (F(1, 18)=12.547, P =0.0023), suggesting that the environmental manipulation affects the power of the left and right gamma oscillations differentially. 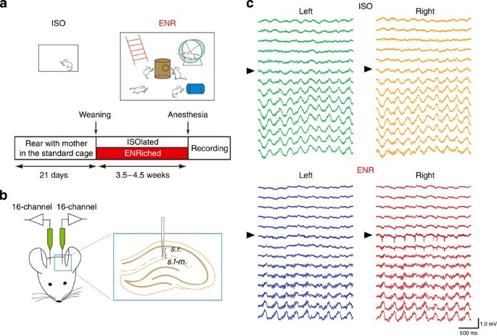Figure 1: Experimental design and recordings from bilateral hippocampi. (a) Experimental design. After weaning at 21 days, rats were reared either individually isolated in standard cages (ISO) or housed together in large enriched cages with wheels and toys (ENR). (b) Recording configuration. Simultaneous left and right CA1in vivorecordings were performed using 16-channel linear silicon probes. (c) Typical recordings of theta-associated gamma oscillations from the entire CA1 area of ISO (upper panel) and ENR (lower panel) rats. Among 16 channels, recordings of 14 channels covering the entire CA1 area (from 200 μm above to 500 μm below pyramidal cell layer; from top traces to the bottom) are shown. Recordings from the pyramidal cell layer are indicated in black triangles. The spacing between channels is 50 μm. Figure 1: Experimental design and recordings from bilateral hippocampi. ( a ) Experimental design. After weaning at 21 days, rats were reared either individually isolated in standard cages (ISO) or housed together in large enriched cages with wheels and toys (ENR). ( b ) Recording configuration. Simultaneous left and right CA1 in vivo recordings were performed using 16-channel linear silicon probes. ( c ) Typical recordings of theta-associated gamma oscillations from the entire CA1 area of ISO (upper panel) and ENR (lower panel) rats. Among 16 channels, recordings of 14 channels covering the entire CA1 area (from 200 μm above to 500 μm below pyramidal cell layer; from top traces to the bottom) are shown. Recordings from the pyramidal cell layer are indicated in black triangles. The spacing between channels is 50 μm. 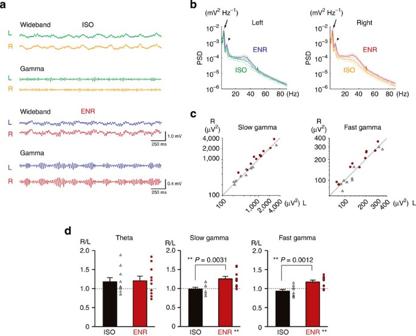Figure 2: Experience-driven emergence of gamma oscillations and left–right asymmetry in CA1s.r. (a) Typical recordings of theta-associated gamma oscillations from the CA1s.r.of ISO (upper panel) and ENR (lower panel) rats at the depth of 200 μm below the pyramidal cell layer. Upper and lower traces depict wideband and gamma band-pass filtered (30–90 Hz) recordings, respectively. L, left; R, right (b) Group averages (solid lines) of power spectrum plots fors.r.recordings. Comparisons were made between ISO and ENR groups of the same side of the hippocampus. The coloured line corresponds to the colour scheme inaandFig. 1c. The averaged power spectral densities (PSDs) were plotted in a logarithmic scale. The dotted lines represent s.e. The peaks for theta and the second harmonic are indicated by arrows and arrowheads, respectively. (c) Left versus right comparisons of slow (30–45 Hz) and fast (55–90 Hz) theta-associated gamma powers. Left (abscissa) versus right (ordinate) theta-associated respective gamma powers are plotted for each recorded rats. Grey triangles and red circles represent ISO and ENR subjects, respectively. The dotted line shows the equilibrium of the left and the right powers. (d) Comparison of right/left (R/L) power ratios ins.r.for theta (3–6 Hz, left panel), slow gamma (middle panel) and fast gamma (right panel) bands. Both slow and fast gamma R/L power ratios significantly exceeded unity (**P<0.01,t-test,NISO=10,NENR=10) in ENR. Both gamma R/L power ratios were also significantly different between ISO and ENR (**P<0.01,t-test,NISO=10,NENR=10). Error bars represent s.e.m. Full size image Figure 2: Experience-driven emergence of gamma oscillations and left–right asymmetry in CA1 s.r. ( a ) Typical recordings of theta-associated gamma oscillations from the CA1 s.r. of ISO (upper panel) and ENR (lower panel) rats at the depth of 200 μm below the pyramidal cell layer. Upper and lower traces depict wideband and gamma band-pass filtered (30–90 Hz) recordings, respectively. L, left; R, right ( b ) Group averages (solid lines) of power spectrum plots for s.r. recordings. Comparisons were made between ISO and ENR groups of the same side of the hippocampus. The coloured line corresponds to the colour scheme in a and Fig. 1c . The averaged power spectral densities (PSDs) were plotted in a logarithmic scale. The dotted lines represent s.e. The peaks for theta and the second harmonic are indicated by arrows and arrowheads, respectively. ( c ) Left versus right comparisons of slow (30–45 Hz) and fast (55–90 Hz) theta-associated gamma powers. Left (abscissa) versus right (ordinate) theta-associated respective gamma powers are plotted for each recorded rats. Grey triangles and red circles represent ISO and ENR subjects, respectively. The dotted line shows the equilibrium of the left and the right powers. ( d ) Comparison of right/left (R/L) power ratios in s.r. for theta (3–6 Hz, left panel), slow gamma (middle panel) and fast gamma (right panel) bands. Both slow and fast gamma R/L power ratios significantly exceeded unity (** P <0.01, t -test, N ISO =10, N ENR =10) in ENR. Both gamma R/L power ratios were also significantly different between ISO and ENR (** P <0.01, t -test, N ISO =10, N ENR =10). Error bars represent s.e.m. Full size image To directly compare left and right gamma power within subjects, we computed the right/left gamma power ratio in each rat in the ISO and ENR groups. The right/left slow gamma power ratio ((R/L) γs ) for ISO rats was 0.987±0.0441 ( P =0.768, t -test; Fig. 2d ), reflecting the balanced left and right hippocampi. Notably, (R/L) γs for ENR was significantly greater than 1 (1.254±0.0649, P =0.00354, t -test; Fig. 2d ), indicating a dominance of gamma oscillation amplitude in the right CA1 s.r. A similar result was obtained with fast gamma ((R/L) γf ); the (R/L) γf for ISO and ENR were 0.935±0.0428 and 1.173±0.0454, respectively, and the (R/L) γf for ENR was significantly greater than 1 ( P =0.0041, t -test). Moreover, both (R/L) γs and (R/L) γf were significantly different between rearing conditions ISO and ENR ((R/L) γs : P =0.00314, t -test; (R/L) γf : P =0.0041, t -test). Together, the ENR condition induces relative increases of the LFP oscillation power on the right side in both the slow and fast gamma range. We next addressed if a shorter housing in ENR can induce similar changes of gamma oscillations. We found that the dominance of the right gamma power was not observed in rats with 1–2 weeks in ENR (at s.r. , (R/L) γs =1.048±0.0943, P =0.828, t -test, N =3; Supplementary Fig. S3 ). This observation is in agreement with previous studies on the kinetics of hippocampal changes after exposure to enriched environments, including increased neurogenesis [9] and enhanced synaptogenesis [6] , [10] . As the gamma oscillations reflect experience-dependent plasticity, we wondered if theta oscillations also undergo analogous changes. Similar spectral analyses were applied for theta (3–6 Hz) oscillations. Surprisingly, there was little effect of rearing condition or side of the hippocampus on theta power (two-way ANOVA; environmental effect: (F(1, 18)=1.528, P =0.232; laterality effect: F(1, 18)=1.817, P =0.194). Notably, we did not detect a significant interaction between the two factors (F(1, 18)=0.129, P =0.7235). The left versus right theta power ratio ((R/L) θ ) of neither ISO nor ENR rats deviated significantly from unity (ISO: 1.178±0.109, P =0.136, N ISO =10; ENR: 1.204±0.122, P =0.127, t -test, N ENR =10; Fig. 2d ). In addition to theta, a power spectral peak in the second harmonic range (6.5–12 Hz) was noticeable ( Fig. 2b , arrows). This second harmonic showed a sign of laterally biased enhancement in ENR rats ( Supplementary Fig. S4 , two-way ANOVA as above, P =0.0374 for environment, P =0.0719 for laterality and P =0.0693 for environment × laterality interaction). These results suggest that possibly the waveform, but not the amplitude, of theta was changed by chronic environmental manipulations. Strong gamma-range oscillations are present in the s.l-m. [2] , a layer characterized by innervation from the entorhinal cortex (that is, the temporoammonic pathway) and the absence of CA3 axons. To examine if the caging animals in ENR has a significant effect on the temporoammonic pathway, we analyzed the theta-associated gamma oscillations in this location. In contrast to the s.r. , the power spectrum density plots of ISO and ENR virtually overlapped in the slow gamma range ( N ISO =9, N ENR =9; Supplementary Fig. S5 ), suggesting that environmental effects on hippocampal CA1 is likely to be mediated by CA3-CA1 synapses. Enhancement of gamma oscillations is NMDAR dependent As NMDAR activation is involved in many forms of CA3-CA1 synaptic plasticity both in vitro and in vivo , we addressed if NMDAR activation is involved in the experience-dependent enhancement of gamma oscillations by administering the NMDAR antagonist ketamine [11] . Rats were reared in ENR for 3–4 weeks, with ketamine included in the drinking water (0.1% w/v, supplemented with 0.5% w/v sucrose; ENR+ket). The ENR+ket rats did not show any apparent behavioural abnormalities ( Supplementary Fig. S6 ). Ketamine administration and laterality showed a significant degree of interaction (two-way ANOVA, F(1, 16)=6.88, P =0.0185). Moreover, the slow gamma power of ENR+ket group was significantly smaller than that of ENR group in both sides (left: P =0.0425, right: P =0.0218, Shaffer’s method, N ENR =10, N ENR+ket =8; Fig. 3a ). The fast gamma, too, showed a significant interaction of ketamine and laterality (F(1, 16)=11.8, P =0.0034). We observed no difference in the (R/L) θ between ENR+ket and ENR ( P =0.734, t -test). In contrast, (R/L) γs in the ketamine-treated rats was significantly lower than ENR rats ( P =0.000455, t -test), and surprisingly shifted below 1 (0.873±0.0528), indicating a left dominance of slow gamma oscillations ( P =0.0472, t -test). Similarly, (R/L) γf for ENR+ket was 0.771±0.0428 ( P =0.0011, t -test) and significantly different from ENR ( P =0.000010, t -test; Fig. 3c ). Acute administration of ketamine (intramuscular injection, 3.0 mg kg −1 ) just before recording in enriched environment-reared rats (ENR+a-ket) did not show the effects of chronic ketamine administration (R/L γs =1.22±0.041, P =0.750, ENR versus ENR+a-ket; R/L γf =1.05±0.044, P =0.137, ENR versus ENR+a-ket, t -test, N ENR+a-ket =4; Fig. 3c ). 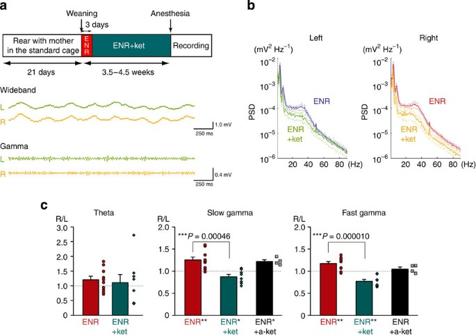Figure 3: Chronic effects of the NMDAR inhibitor ketamine on the theta state power spectrum. (a) Experimental design and CA1s.r.theta LFP recordings. After weaning at postnatal day 21, rats were reared in ENR for 3 days to learn to drink from water bottles. Thereafter, the water was supplemented with ketamine (0.1% w/v) until the day of the recording (upper panel). Typical recording of bilateral theta-associated gamma oscillations from the CA1s.r.of an ENR+ketamine (ENR+ket) rat. Left (L) and right (R) paired traces are wideband and slow gamma-filtered recordings, respectively (lower panel). (b) PSDs of the left and right CA1s.r.theta state LFPs in ENR and ENR+ket conditions. The averaged PSDs were plotted as inFig. 2b. (c) Mean R/L power ratios of theta (left panel), slow gamma (middle panel) and fast gamma (right panel) in CA1s.r.of ENR and ENR+ket rats. The slow and fast gamma power ratios of ENR+ket were significantly lower than 1 (*P<0.05 and **P<0.01, respectively,t-test,NENR=10,NENR+ket=8). The ENR and ENR+ket power ratios were significantly different (***P<0.001,t-test,NENR=10,NENR+ket=8). Acute effect (within 90 min) of intramuscular ketamine administration (3.0 mg kg−1, ENR+a-ket,NENR+a-ket=4) on slow and fast gamma power is also shown in black in the middle and the right panel. ENR+a-ket did not show the inhibitory effects seen in ENR+ket. Error bars represent s.e.m. Figure 3: Chronic effects of the NMDAR inhibitor ketamine on the theta state power spectrum. ( a ) Experimental design and CA1 s.r. theta LFP recordings. After weaning at postnatal day 21, rats were reared in ENR for 3 days to learn to drink from water bottles. Thereafter, the water was supplemented with ketamine (0.1% w/v) until the day of the recording (upper panel). Typical recording of bilateral theta-associated gamma oscillations from the CA1 s.r. of an ENR+ketamine (ENR+ket) rat. Left (L) and right (R) paired traces are wideband and slow gamma-filtered recordings, respectively (lower panel). ( b ) PSDs of the left and right CA1 s.r. theta state LFPs in ENR and ENR+ket conditions. The averaged PSDs were plotted as in Fig. 2b . ( c ) Mean R/L power ratios of theta (left panel), slow gamma (middle panel) and fast gamma (right panel) in CA1 s.r. of ENR and ENR+ket rats. The slow and fast gamma power ratios of ENR+ket were significantly lower than 1 (* P <0.05 and ** P <0.01, respectively, t -test, N ENR =10, N ENR+ket =8). The ENR and ENR+ket power ratios were significantly different (*** P <0.001, t -test, N ENR =10, N ENR+ket =8). Acute effect (within 90 min) of intramuscular ketamine administration (3.0 mg kg −1 , ENR+a-ket, N ENR+a-ket =4) on slow and fast gamma power is also shown in black in the middle and the right panel. ENR+a-ket did not show the inhibitory effects seen in ENR+ket. Error bars represent s.e.m. Full size image Interhemispheric gamma coherence is elevated in ENR As a significant portion of CA1 s.r. innervation originates from the contralateral CA3 [12] , we next investigated the bilateral organization of oscillatory activities. To this end, we first calculated the cycle-by-cycle phase difference of the left and right CA1 s.r. gamma oscillations. The phase-difference histograms of slow gamma are plotted for an ISO rat and an ENR rat in Fig. 4a . The distribution for the ENR example has a smaller circular s.d., suggesting a more tightly coupled temporal coordination of bilateral gamma oscillations than ISO. To compute the phase relationship across all frequency ranges, we computed the magnitude squared coherence of bilateral LFPs during theta states for both ISO and ENR rats ( Fig. 4b ). Previous studies have demonstrated that theta, but not gamma, oscillations are highly coherent across hemispheres [13] , and our results confirmed this with a high mean interhemispheric CA1 s.r. theta coherence for both ISO and ENR groups (ISO: 0.799±0.022, N ISO =10; ENR: 0.824±0.024, N ENR =10). As reported, we also found overall lower coherence in the slow gamma band, but it was significantly higher in the ENR group than in the ISO group (0.430±0.0425 versus 0.231±0.0474, respectively, P =0.00583, t -test). In the ISO rats, the interhemispheric coherence was below 0.3 across the slow gamma band, indicating a desynchronized phase relationship between the hemispheres. In contrast, the coherence was prominently elevated in ENR, reaching a peak value of approximately 0.5 at ~36 Hz ( Fig. 4b ), suggesting that the synaptic inputs to both sides of CA1 are temporally more coordinated in ENR. In both ISO and ENR, the coherence was low in the fast gamma range and beyond. The gamma coherence enhancement for ENR was also seen for s.l-m. recordings, although to a smaller degree than s.r. ( Figs 4c and 5b ). Chronic treatment with ketamine (ENR+ket) significantly decreased the interhemispheric coherence (0.231±0.0529, P =0.00887, t -test; Fig. 4d ). Interestingly, the second harmonic of theta showed a significant higher coherence in ENR (ISO: 0.497±0.0356, ENR: 0.667±0.0269, P =0.0013, t -test, N ISO =10, N ENR =10; Supplementary Fig. S4b ). We also observed the laterally biased increase of gamma power and coherence in the stratum oriens ( s.o. ) ( Fig. 5a ), although it should be noted that the power of gamma is visibly smaller than that of s.r. Indeed, the average powers of gamma oscillations at s.o. (−200 μm from the pyramidal cell layer) were 20.3% and 13.9% of those of s.r. (+200 μm) in ISO and ENR, respectively. 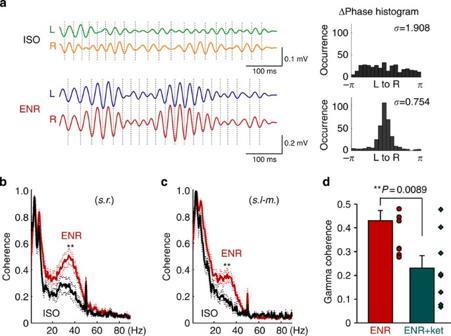Figure 4: Interhemispheric gamma coherence is higher in ENR. (a) Example traces of simultaneously measured left (L) and right (R) CA1s.r.slow gamma oscillations in different rearing conditions. Dotted lines indicate the bottom peak of right-side gamma oscillations. The interhemispheric gamma phase was computed for each gamma cycle by Hilbert transformation, and circularly subtracted to obtain the phase difference. The phase-difference histograms of gamma LFPs for 10 s are plotted in the right panels. Theσvalue denotes the circular s.d. (b) Interhemispheric coherence spectrum of ISO (black) and ENR (red) in CA1s.r. There is a significant difference between ISO and ENR in the gamma range (**P<0.01,t-test,NISO=10,NENR=10). (c) Similar plot as (b) in CA1s.l-m. There is a significant difference between ISO and ENR (**P<0.01,t-test,NISO=10,NENR=10) in the slow gamma range. (d) Interhemispheric slow gamma coherence comparison of ENR versus ENR+ket (**P<0.01,t-test,NENR=10,NENR+ket=8). Each dot represents an animal. Error bars represent s.e.m. Figure 4: Interhemispheric gamma coherence is higher in ENR. ( a ) Example traces of simultaneously measured left (L) and right (R) CA1 s.r. slow gamma oscillations in different rearing conditions. Dotted lines indicate the bottom peak of right-side gamma oscillations. The interhemispheric gamma phase was computed for each gamma cycle by Hilbert transformation, and circularly subtracted to obtain the phase difference. The phase-difference histograms of gamma LFPs for 10 s are plotted in the right panels. The σ value denotes the circular s.d. ( b ) Interhemispheric coherence spectrum of ISO (black) and ENR (red) in CA1 s.r . There is a significant difference between ISO and ENR in the gamma range (** P <0.01, t -test, N ISO =10, N ENR =10). ( c ) Similar plot as ( b ) in CA1 s.l-m . There is a significant difference between ISO and ENR (** P <0.01, t -test, N ISO =10, N ENR =10) in the slow gamma range. ( d ) Interhemispheric slow gamma coherence comparison of ENR versus ENR+ket (** P <0.01, t -test, N ENR =10, N ENR+ket =8). Each dot represents an animal. Error bars represent s.e.m. 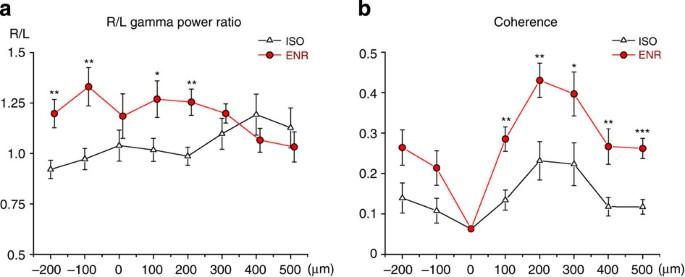Figure 5: Recording site-dependence of interhemispheric slow gamma relationship. (a) Depth profile of R/L ratio of slow gamma power. The pyramidal cell layer is the reference point, and positive values of distance indicate directions towardss.l-m.(b) Depth profile of interhemispheric slow gamma coherence. (*P<0.05, **P<0.01 and ***P<0.001 show the statistical significance between ISO versus ENR, respectively (t-test,NISO=8 for depth −200, 10 for depth −100 to 300, 9 for depth −400 and 500;NENR=10 for depth −200 to 200, 9 for depth 400 and 500). Error bars represent s.e.m. Full size image Figure 5: Recording site-dependence of interhemispheric slow gamma relationship. ( a ) Depth profile of R/L ratio of slow gamma power. The pyramidal cell layer is the reference point, and positive values of distance indicate directions towards s.l-m. ( b ) Depth profile of interhemispheric slow gamma coherence. (* P <0.05, ** P <0.01 and *** P <0.001 show the statistical significance between ISO versus ENR, respectively ( t -test, N ISO =8 for depth −200, 10 for depth −100 to 300, 9 for depth −400 and 500; N ENR =10 for depth −200 to 200, 9 for depth 400 and 500). Error bars represent s.e.m. Full size image Synapse density increases in the right CA1 s.r. in ENR To investigate the anatomical correlates of this experience-dependent induction of LFP enhancement, the organization of glutamatergic and GABAergic synapses in CA1 was examined by immunofluorescent labelling in a separate set of rats ( Fig. 6a , Supplementary Fig. S7 ). We used immunofluorescence labelling for vesicular glutamate transporter type 1 (VGLUT1) and vesicular GABA (γ-aminobutyric acid) transporter (VGAT) to label axon terminals of glutamatergic and GABAergic synapses, respectively. Confocal imaging of immunolabelled CA1 s.o. (VGLUT1: N ISO =4, N ENR =6; VGAT: N ISO =3, N ENR =4), s.r. ( N =5, 9; 6, 8) and s.l-m. ( N =5, 5; 6, 6) revealed punctate distributions of VGLUT1 and VGAT. Two-way ANOVA analysis indicated that the R/L balance of mean VGLUT1 fluorescence intensity is higher in ENR (F(1, 28)=7.24, P =0.0119; Fig. 6b ) and is dependent on the anatomical location (F(2, 28)=4.51, P =0.02). Moreover, a significant degree of interaction between rearing condition and anatomical location was revealed (F(2, 28)=3.55, P =0.0423). The R/L balance of fluorescence intensity was also examined for VGAT signals and housing environment, and a weaker but significant interaction was detected (F(1, 27)=4.51, P =0.0429; Supplementary Fig. S7b ). The two-way ANOVA analysis suggests that rearing condition is a significant factor that influences the R/L balance of VGAT-positive terminals (F(1, 27)=4.51, P =0.0249). Furthermore, using confocal microscopy, we counted the fluorescent puncta in respective images. The R/L balances of puncta were similar to those of fluorescence intensity for VGLUT1 and VGAT ( Supplementary Fig. S7c ). Next, we examined the CA1 s.r. spine synapse density by electron microscopy ( Fig. 6c ). In ISO rats, the average spine densities of the left and the right s.r. were 1.30±0.07 and 1.31±0.07 spines per μm 3 , respectively ( Fig. 6d ). However, in ENR rats, the spine density of the right was approximately twice of the left (0.831±0.0824 versus 1.96±0.0959, spines per μm 3 ; paired t -test, P =0.00998). Despite these differences in spine density, the distribution of postsynaptic density areas could not be distinguished by either laterality or rearing condition ( Supplementary Fig. S8 ). 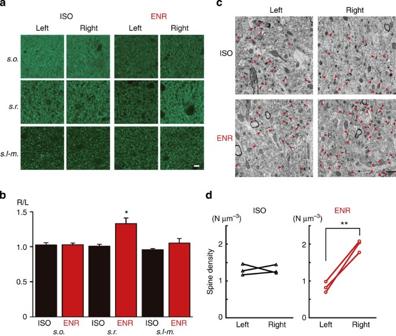Figure 6: Asymmetrical increase of synapse numbers in CA1s.r.in ENR. (a) Immunostaining of glutamatergic presynaptic terminals by VGLUT1. Typical images of VGLUT1 immunostaining (upper panel). VGLUT1 was used to label excitatory presynaptic terminals. Each image is a maximum intensity projection of seven consecutive depth images (150 μm interval). Note that VGLUT1 immunoreactivity is more intense in thes.r. of the ENR rat. Scale bar, 10 μm. (b) Bar graphs of the left versus right fluorescence intensity balance for VGLUT1. The mean VGLUT1 fluorescence intensity was more intense in the CA1s.r. of the ENR rat (*P<0.05, Tukey’s honestly significant difference test,NISO=4,NENR=6 (s.o.);NISO=5,NENR=9 (s.r.);NISO=5,NENR=5 (s.l-m.)). (c) Representative EM images of the left and right CA1s.r. prepared from ISO and ENR rats. Scale bar, 1.0 μm. Arrowheads indicate the locations of postsynaptic density thickening. (d) Pairwise comparisons of left versus right spine density in CA1s.r.Three rats were investigated for each rearing condition (**P<0.01, pairedt-test,NISO=3,NENR=3). Error bars represent s.e.m. Figure 6: Asymmetrical increase of synapse numbers in CA1 s.r. in ENR. ( a ) Immunostaining of glutamatergic presynaptic terminals by VGLUT1. Typical images of VGLUT1 immunostaining (upper panel). VGLUT1 was used to label excitatory presynaptic terminals. Each image is a maximum intensity projection of seven consecutive depth images (150 μm interval). Note that VGLUT1 immunoreactivity is more intense in the s.r . of the ENR rat. Scale bar, 10 μm. ( b ) Bar graphs of the left versus right fluorescence intensity balance for VGLUT1. The mean VGLUT1 fluorescence intensity was more intense in the CA1 s.r . of the ENR rat (* P <0.05, Tukey’s honestly significant difference test, N ISO =4, N ENR =6 ( s.o. ); N ISO =5, N ENR =9 ( s.r. ); N ISO =5, N ENR =5 ( s.l-m. )). ( c ) Representative EM images of the left and right CA1 s.r . prepared from ISO and ENR rats. Scale bar, 1.0 μm. Arrowheads indicate the locations of postsynaptic density thickening. ( d ) Pairwise comparisons of left versus right spine density in CA1 s.r. Three rats were investigated for each rearing condition (** P <0.01, paired t -test, N ISO =3, N ENR =3). Error bars represent s.e.m. Full size image In the present study, we find that chronic exposure to the ENR condition enhances gamma oscillations in CA1 s.r. of the right hippocampus. To our knowledge, this is the first demonstration of in vivo neural oscillation changes in the hippocampus by ENR. The anesthetized condition provides a stable resting oscillatory pattern without external stimuli, and therefore reflects internally driven rhythms. Under similar conditions, gamma oscillations in hippocampal CA3 have been demonstrated to represent balanced excitatory and inhibitory synaptic currents [14] . Our results support this idea, as right-biased enhancements occur in both glutamatergic and GABAergic terminal immunolabelling in ENR. Hippocampal CA1 area receives two distinct gamma-modulated inputs: (1) the fast gamma (>65 Hz) driven by the temporoammonic pathway and localized in the s.l-m. and (2) the slow gamma (<50 Hz) conveyed by the CA3-CA1 input and localized in s.r. [7] As most of the synaptic inputs in CA1 s.r. originate from bilateral CA3 pyramidal cells [12] , CA3-CA1 synapses are likely to be involved in this change. Under urethane anesthesia, theta oscillations are sensitive to atropine, a blocker of muscarinic receptors [15] , [16] . Interestingly, muscarinic receptors have been reported to mediate gamma oscillations in the hippocampus [17] and are more densely distributed in the right hippocampus in rats [18] . Moreover, rats reared in ENR express higher cortical and hippocampal levels of nerve growth factor transcript, a neurotrophin important for development and maintenance of cholinergic neurons [19] . Although lateralized cholinergic activity is yet to be shown, it is tempting to speculate that increased cholinergic transmission combined with the laterally biased distribution of muscarinic receptors contributes to the gamma-activity enhancement. Recent studies have revealed that several mechanisms of ENR induced changes in CA1 pyramidal cells, including increased expression of the microtubule motor protein KIF17 that traffics NMDARs [10] , and changes in the active membrane properties of CA1 pyramidal cells, resulting in a lower action potential discharge threshold and more depolarized action potential-induced after-hyperpolarization potential [20] . Such membrane property changes or extrasynaptic NMDARs [21] may also provide mechanisms for synaptic input-dependent enhancement of gamma oscillations. Although tissue impedance increase due to increase in spine density is a potential cause of the LFP gamma-amplitude enhancement, our result showing specific enhancement of gamma-band coherence proposes that the temporal coordination of interhemispheric neural dynamics is indeed strengthened by ENR. Lateralization of brain function is distinct in higher primates and humans [22] . As for memory processing, the use of the right hippocampus is dominant during spatial memory tasks [23] , [24] , whereas episodic memory is more associated with the left hippocampus [24] , [25] . The significance of the right hippocampus in spatial memory is apparent in rodents as well. For example, mRNA expression changes associated with spatial learning predominantly occur in the right hippocampus, [26] and split-brain mice perform better in the Barnes maze when the right hippocampus is preferentially used [27] . Moreover, asymmetrical circuit formation in rodent hippocampus has previously been identified in terms of differential glutamatergic receptor subunit distribution [28] , [29] , [30] . Such circuit formation is partly due to a genetic program, although the exact mechanism is yet to be identified [31] . Experience-dependent enhancement of bilateral gamma oscillations provides an additional mechanism for this brain lateralization. Experience-dependent enhancement of hippocampal asymmetry may underlie the mechanisms behind highly lateralized brain functions in higher mammals, as multiple human functional magnetic resonance imaging studies report that the hippocampus and surrounding regions are critical for setting the lateralization of cortical language-processing areas [32] , [33] , [34] . Although the specific molecular mechanism is yet to be addressed, the ENR-induced changes in CA1 are found to be NMDAR dependent and reflected in the spine density, hinting at a mechanism similar to classical long-term potentiation. It is conceivable that lateralized synaptogenesis is a hallmark of the maturation of hippocampal circuitry in response to environmental enrichment. Rearing environments All procedures involving animal care, surgery and sample preparation were approved by the Animal Experimental Committee of RIKEN Brain Science Institute and performed in accordance with the guidelines of the Animal Experimental Committee of RIKEN Brain Science Institute. Male Long-Evans rats were weaned at postnatal 21 days. For the ISO group, rats were caged individually after weaning and raised in standard cages (42 (l) × 20 (w) × 21 (h) cm 3 ). For the ENR group, 6–8 littermate rats were housed together in a large cage (74 × 36 × 35 cm 3 ) with running-wheels, tunnels and toys, whose locations were changed twice a week. In both housing environments, water and food were given ad libitum . For chronic ketamine treatment in ENR (ENR+ket), the rats were given normal water for the first 3 days immediately after weaning to learn to drink from the facility bottles. Thereafter, ketamine (0.1% w/v) and sucrose (0.5% w/v, to counter the taste of ketamine) were introduced in the drinking water so that the average intake of the fluid would result in a chronic plasma concentration of 3 mg kg −1 ketamine. Considering the liver metabolism [35] and the frequency of water intakes [36] , the average plasma concentration of ketamine is calculated to be an order of magnitude smaller than the dosage reported to be effective as antidepressant in rats [11] . The amounts of consumed water by ENR and ENR+ket rats were not significantly different. Electrophysiological and anatomical studies were performed 3.5–4.5 weeks after rearing in the designated environments. LFP recording Bilateral LFP recordings were performed using 16-channel linear silicon probes (50 μm inter-recording site interval; Alx15-5mim-50-177-A16; NeuroNexus, Ann Arbor, MI). The tip of the silicon probe was dipped into a DiI solution (8 mg DiI in 1 ml acetone) to mark the electrode penetration by fluorescence for post-hoc verification. Rats were anesthetized with urethane (1.6 g kg −1 ) by intraperitoneal (i.p.) administration and fixed in a stereotaxic apparatus (Kopf, Tujunga, CA, USA). The body temperature of the animals was maintained at 37 °C using a heat pad with feedback temperature controller (TR-200; FST, Foster City, CA, USA). Two small craniotomies of 1.0 mm diameter were made at stereotaxic locations of anterior-posterior (AP) −3.0 mm and medial-lateral (ML) ±2.3 mm from the bregma so that they are above the bilateral dorsal hippocampal CA1. After removing the dura mater, a 16-channel linear silicon probe was inserted vertically into the centre of the craniotomy on each side. The location of the recording site at the CA1 pyramidal layer was recognized by (1) the depth of the probe, (2) the emergence of the typical sharp wave-associated ripples (>100 Hz) and (3) the presence of multi-unit activity. The depths of the silicon probes were adjusted to the same level in every recording session. The signals were buffered by a HS-27 head-stage preamplifier (Neuralynx, Bozeman, MT, USA), which were then digitized with a Digital Lynx system (Neuralynx) at a sampling rate of ~32.556 kHz and a bandwidth of 0.1–9000 Hz. Typically, recordings were made 2 –6 h after the induction of anesthesia. A volume of 1.5–2.0 ml physiological saline (0.9% NaCl) with 5% glucose was supplied (i.p.) at 1.5–2 h intervals. After the recording session, the rat was deeply anesthetized with additional urethane and transcardially perfused by saline followed by 4.0% paraformaldehyde in 0.1 M phosphate buffer (pH 7.4). Serial coronal sections measuring 60 μm were cut using a vibratome (PRO 7; Dosaka, Kyoto, Japan) for electrode track verification. Experiments with mismatching recording sites were excluded from analyses. LFP data analysis Data processing was done on a Linux workstation running custom programs written in Matlab and Perl. For LFP analysis, the wideband recordings were down-sampled at 1,250 Hz. Theta periods were detected by first computing the spectrogram (window size=1 s, overlap=0.5 s) and finding the intervals that satisfy the following two criteria: (1) The ratio of the peak powers of the theta band (3.5–7 Hz) and the delta (2-3 Hz) band in each bin exceeds 0.6. (2) The length of the interval is at least 15 s long. For spectral power analyses, PSD was estimated by the Welch periodogram method using a Hamming window (window size=1.64 s; overlap=0.82 s). Theta and gamma powers were computed by integrating the PSD for 3–6, 30–45 and 55–90 Hz, respectively. The average spectral power was first calculated per animal over multiple recording sessions and treated as a discrete sample value for further statistical comparisons (such as left versus right or ENR versus ISO). The amplifier gains were calibrated by passing sinusoidal signals of various frequencies with a signal generator and recording them in saline solution ( Supplementary Fig. S1 ). To calculate a phase-difference histogram, the LFPs were first filtered using zero-phase digital filtering with a Butterworth filter (order=3, pass band=30–45 Hz). The Hilbert transform was then applied to the filtered LFP to find the instantaneous phase at each time point. Phase-difference histogram was calculated by collecting the instantaneous phase of the left LFP when the right-channel gamma phase is at the bottom peak. For display purposes, the histogram was circularly permutated so that the mode of the distribution is aligned at the centre. The circular mean is calculated as the vector average of the phases in the polar coordinate, and the circular s.d. was calculated as , where R is the norm of the vector average of the phases. The coherence between the two LFP signals x ( t ) and y ( t ) was computed using the ‘mscohere’ function in MatLab that computes: , where P xy ( f ) denotes the cross-power spectral density of the signals x and y at frequency f , that is, . E {·} denotes the expected value operator. Error bars in all figures and Supplementary Materials represent the s.e.m. Immunohistochemistry Rat brains were fixed with 4.0% paraformaldehyde, and coronal slices (40 μm) were prepared. After blocking in TBS containing 3% BSA and 0.1% Trinton X-100 for 1 h, the sections were incubated with primary antibodies (VGLUT1, 1:500, VGluT1-Rb-Af500, VGAT, 1:500, VGAT-GP-Af1000; Frontier Institute, Ishikari, Japan) for overnight in TBS with 1% BSA containing 0.1% Triton X-100. Signals were visualized by incubation with Alexa 488 and 594 conjugated secondary antibodies (Life technologies, Grand Island, NY, USA) for 2 h. Immunolabelled sections were examined using a FV1000 confocal microscope (Olympus, Tokyo, Japan). Confocal images (42 × 42 μm 2 , 1,024 × 1,024 pixels, 150 nm z-stack interval) were taken with a × 60 oil immersion lens (numerical aperture=1.42). Seven consecutive depth images close to the surface were used for analysis. For the analysis of fluorescence intensity balance, the pixel values of the seven images were summed, and the background of each image was subtracted. The background was computed as the mean of the 100 smallest pixel values in a given image. For the analysis of puncta density, bright punctate spots of 250–1,500 nm diameter were counted. Large hollow structures (for example, blood vessels and neuronal somata) were avoided. On average, the density was computed from an area of~600 μm 2 per sample. Electron microscopy Rats were deeply anesthetized with urethane (i.p.>2.5 g kg −1 ) and transcardially perfused by 0.1 M PBS, followed by perfusion with a fixative (4.0% paraformaldehyde, 0.1% glutaraldehyde and 15% saturated picric acid in 0.1 M phosphate buffer, 250 ml). Following overnight postfixation at 4 °C, 60 μm sections were prepared from the dorsal hippocampus of the identical stereotaxic coordinate to the electrophysiological recording. Special care was taken to match the left and the corresponding right hippocampal sections of the same animal. Ultra-thin sections were prepared in the same method described elsewhere (Shinohara PNAS 2008). Ultra-thin serial sections were examined using a Tecnai F12 electron microscope (FEI, Hillsboro, OR) equipped with a TemCam-F416 digital camera (TVIPS, Gauting, Germany; 16 mega-pixels). Images were taken at a magnification of × 4,800. Morphological analyses The spines of CA1 pyramidal cell apical dendrites (at ~200 μm distant from the centre of the pyramidal cell layer) were analyzed. For postsynaptic density area analysis, a merged image of size 16 × 16 μm 2 were constructed from 3 × 3 adjacent images by the ‘photomerge’ function of Photoshop (Adobe, San Jose, CA). All the spine-type pyramidal cell synapses in this area that were contained completely within the serial depth image stack were analyzed. The postsynaptic density area was quantified as the summation of the postsynaptic density lengths of a spine in the serial image stack multiplied by the thickness of the stack (60 nm). The area of the spines more than 130 was analyzed. For spine density estimation, the dissector method [37] was used. Briefly, a pair of long s.r. serial sections (~200 μm distant from the pyramidal cell layer, 9 × 150~200 μm 2 ; along the mediolateral direction of the coronal section) were compared and only synapses that were found in the first image but not appeared in the second were counted. The spine density was computed as the spine count divided by the product of the image area and the thickness of the section (60 nm). Counting was done in the opposite direction of serial sections as well, and averaged. How to cite this article: Shinohara, Y. et al . Experience enhances gamma oscillations and interhemispheric asymmetry in the hippocampus. Nat. Commun. 4:1652 doi: 10.1038/ncomms2658 (2013).